Megakaryocyte-specific Profilin1-deficiency alters microtubule stability and causes a Wiskott–Aldrich syndrome-like platelet defect Wiskott–Aldrich syndrome (WAS) is caused by mutations in the WAS gene and is characterized by immunodeficiency, eczema and microthrombocytopenia. The molecular link between WAS mutations and microthrombocytopenia is unknown. Profilin1 (Pfn1) is a key actin-regulating protein that, besides actin, interacts with phosphoinositides and multiple proline-rich proteins, including the WAS protein (WASp)/WASp-interacting protein (WIP) complex. Here we report that mice with a megakaryocyte/platelet-specific Pfn1 deficiency display microthrombocytopenia due to accelerated turnover of platelets and premature platelet release into the bone marrow. Both Pfn1-null mouse platelets and platelets isolated from WAS patients contained abnormally organized and hyperstable microtubules. These results reveal an unexpected function of Pfn1 as a regulator of microtubule organization and point to a previously unrecognized mechanism underlying the platelet formation defect in WAS patients. Blood platelets are anucleated cell fragments derived from highly polyploid, mature bone marrow (BM) megakaryocytes (MKs) that convert their cytoplasm by a cytoskeleton-driven process into long protrusions (proplatelets). These proplatelets extend into the blood stream where shear forces release the so-called pre-platelets, and final platelet shaping and sizing occurs [1] . Wiskott–Aldrich syndrome (WAS) is a X-linked disease caused by mutations in the WAS gene and is characterized by immunodeficiency, eczema and severe thrombocytopenia with reduced mean platelet volume (microthrombocytopenia) [2] . The WAS protein (WASp) is an important regulator of actin assembly [3] and is constitutively associated with the WASp-interacting protein (WIP) in resting and activated platelets to prevent its degradation [4] , [5] . WASp-deficient mice display premature platelet release into the BM but only a moderate thrombocytopenia with normal-sized platelets [6] , [7] . Similarly, a patient carrying a mutation in the WIP gene [8] or WIP-deficient mice that also lack WASp in platelets have an unaltered platelet size and suffer from a thrombocytopenia partially caused by increased platelet clearance [5] , [9] . The reason for the discrepancy in platelet phenotypes between WAS patients and WASp-deficient mice remains enigmatic and the molecular link between WAS mutations and microthrombocytopenia is unknown. Another key regulator of actin turnover is the small (15 kDa) protein, Profilin1 (Pfn1) that binds to monomeric G-actin, thereby accelerating the nucleotide-exchange from ADP to ATP and consequently promoting actin filament elongation [10] . In mammals, four different Pfn isoforms have been identified. Pfn1 is ubiquitously expressed with the exception of muscle tissue. Pfn2 is highly expressed in the central nervous system, whereas Pfn3 and 4 are predominantly found in the testis [11] . Pfn1 is essential for early development as Pfn1-null embryos die at the two-cell stage due to defective cell division [12] . Besides its actin-binding domain, Pfn1 is endowed with a domain that binds to phosphoinositides, which in turn affects actin and ligand binding, as well as PLCγ1 activity [11] , [13] . In addition, the poly- L -proline-binding domain, which is required for the interaction with multiple proline-rich proteins, is involved in various cellular processes, such as membrane trafficking, focal contact formation, signalling and actin dynamics [11] . Moreover, Pfn1 interacts with N-WASp [14] and can be bound by glutathione S -transferase–WIP in mammalian cells [15] . However, the significance of these interactions is not known. Here we report that mice with a MK/platelet-specific Pfn1 deficiency display a microthrombocytopenia and premature platelet release into the BM, thereby reproducing a central hallmark of WAS in humans. Pfn1-deficient platelets contained misarranged and hyperstable microtubules, a defect that was also found in platelets from WAS patients. Taken together, these results reveal an unexpected function of Pfn1 as a regulator of microtubule organization and point to a previously unrecognized mechanism underlying the platelet formation defect in WAS patients. Pfn1 fl/fl, Pf4-Cre mice recapitulate key features of the WAS We assessed Pfn expression in murine platelets by reverse transcription–PCR, which yielded a Pfn1 band at 305 bp, whereas other Pfn isoforms were not detected ( Supplementary Fig. 1a ). To investigate the role of Pfn1 in MKs and platelets, we engineered Profilin1 fl/fl, Pf4-Cre mice (further referred to as Pfn1 −/− ) that lack Pfn1 expression specifically in MKs and platelets. Complete loss of Pfn1 in mutant platelets ( Supplementary Fig. 1b ) and BM MKs ( Supplementary Fig. 1c ) was confirmed by western blot analysis. Pfn1 −/− mice (12 weeks old) displayed a microthrombocytopenia with a reduction in platelet count of ~40% ( Fig. 1a ) and on average smaller-sized platelets ( Fig. 1b , forward scatter signal) with a highly variable and frequently very thin platelet shape ( Fig. 1c ). Analysis of platelet area on transmission electron microscopic (TEM) images ( Fig. 1d ) and blood smears ( Supplementary Fig. 2 ) confirmed the reduced size of platelets in Pfn1 −/− mice. This microthrombocytopenia was also observed in 6-week-old mice and thus appeared to be an age-independent phenotype ( Supplementary Fig. 3a ). Of note, heterozygous mice displayed normal platelet counts but still significantly smaller platelets, albeit not as pronounced as in Pfn1 −/− mice ( Supplementary Fig. 3b ). The expression of prominent surface proteins of Pfn1 −/− platelets (12-week-old mice) was markedly reduced most probably due to the smaller platelet size ( Supplementary Fig. 3c ), whereas the distribution of α- and dense granules was not affected by the reduced platelet size (1.53±1.01 granules per μm 2 in controls versus 1.51±0.93 granules per μm 2 in Pfn1 −/− platelets). Thus, Pfn1 −/− mice represent the first mouse model of microthrombocytopenia, a hallmark of WAS in humans [2] , which could not be reproduced in WASp- or WIP-deficient mice [6] , [16] . 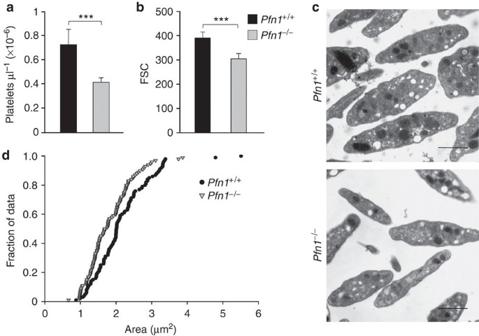Figure 1: Microthrombocytopenia inPfn1−/−mice. (a,b) Fluorescence-activated cell sorter analyses. (a) Peripheral platelet counts. (b) Platelet size. FSC indicates forward scatter. Values are mean±s.d. (n=6 versus 6). (c) TEM analysis of resting platelets. Scale bar, 1 μm. (d) Measurement of platelet area by means of TEM images. Unpaired Student’st-test: ***P<0.001. Figure 1: Microthrombocytopenia in Pfn1 −/− mice. ( a , b ) Fluorescence-activated cell sorter analyses. ( a ) Peripheral platelet counts. ( b ) Platelet size. FSC indicates forward scatter. Values are mean±s.d. ( n =6 versus 6). ( c ) TEM analysis of resting platelets. Scale bar, 1 μm. ( d ) Measurement of platelet area by means of TEM images. Unpaired Student’s t -test: *** P <0.001. Full size image Pfn1 −/− mice had a strongly decreased in vivo platelet life span ( Fig. 2a , T 1/2 of control platelets: 58.4 h, T 1/2 of Pfn1 −/− platelets: 24.7 h). Of note, splenectomy had no long-term effect on platelet counts in Pfn1 −/− mice ( Fig. 2b ). However, depletion of macrophages with clodronate-encapsulated liposomes strongly increased platelet counts in Pfn1 −/− mice, indicating that macrophages preferentially remove Pfn1 −/− platelets from the circulation ( Fig. 2c ). The mice did not develop splenomegaly ( Supplementary Fig. 4a ), but the plasma thrombopoietin (TPO) levels as well as the number of MKs in the spleen and BM were moderately increased, which is consistent with the current reciprocal model of circulating plasma TPO concentration to MK/platelet mass ( Supplementary Fig. 4a ). Furthermore, the ploidy of BM MKs was slightly elevated in the mutant animals ( Supplementary Fig. 4b ), which is indicative of an increased proportion of mature MKs. The ultrastructure of Pfn1-null BM MKs revealed similarities to that of WASp-null MKs [7] . Pfn1-null BM MKs either could be categorized as (I) MKs with normally distributed granules and a well-developed demarcation membrane system ( Fig. 3a , lower left), a membrane reservoir for future platelets, or as (II) MKs with signs of fragmentation ( Fig. 3a , lower and upper right). Immunostaining on BM cross-sections of intact femora ( Fig. 3b and Supplementary Fig. 4c ) and intravital two-photon microscopy (dashed arrows in Fig. 3c and Supplementary Videos 1 and 2 ) confirmed that the majority of Pfn1 −/− MKs released platelets into the BM compartment next to the sinusoids, a defect that is also seen in WASp-deficient mice, although to a lesser extent ( Supplementary Fig. 13a and ref. 7 ). This premature platelet release seemed not to be caused by defective proplatelet formation as revealed by two-photon microscopy (arrow in Supplementary Video 2 ) and in an in vitro proplatelet formation assay ( Supplementary Fig. 4a ), nor to an aberrant localization of MKs within the BM ( Supplementary Fig. 4d ). Podosomes, F-actin-rich matrix contacts, have been proposed as an indicator of MK motility and the ability to extend proplatelets through the basal membrane into the blood stream [17] . To test podosome formation in MKs, we allowed them to spread on a collagen I matrix and stained for F-actin-rich podosomes ( Fig. 3d ) and for p-ASAP, WASp or vinculin, as podosomal markers ( Supplementary Fig. 5 ). Pfn1 −/− MKs barely formed podosomes as compared with control MKs. In addition, mutant MKs spread on fibrinogen contained an enormous amount of acetylated tubulin, which has been associated with increased microtubule stability ( Supplementary Fig. 4e ) [18] . These results suggested that the thrombocytopenia in Pfn1 −/− mice is caused by both accelerated platelet clearing by macrophages and the premature platelet release into the BM due to altered cytoskeletal dynamics, and consequently impaired proplatelet extension through the basal membrane. 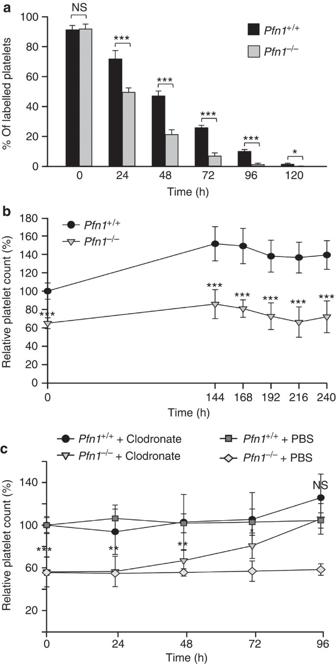Figure 2: Altered platelet survival inPfn1−/−mice. (a) Platelet life span was measured by injection of DyLight 488 α-GPIX. Values are mean±s.d. (n=5 versus 5). Platelet counts were monitored over time after (b) splenectomy and (c) clodronate-encapsulated liposome-mediated macrophage depletion. Unpaired Student’st-test: *P<0.05; **P<0.01; ***P<0.001; NS, non-significant. Figure 2: Altered platelet survival in Pfn1 −/− mice. ( a ) Platelet life span was measured by injection of DyLight 488 α-GPIX. Values are mean±s.d. ( n =5 versus 5). Platelet counts were monitored over time after ( b ) splenectomy and ( c ) clodronate-encapsulated liposome-mediated macrophage depletion. Unpaired Student’s t -test: * P <0.05; ** P <0.01; *** P <0.001; NS, non-significant. 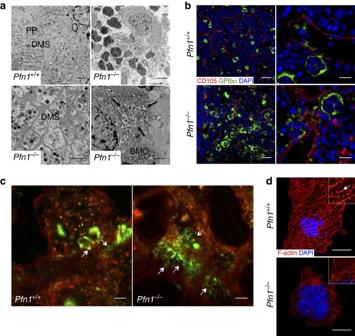Figure 3: Premature platelet release into BM compartment. (a) TEM analysis of BM MKs (upper left: control MK). Scale bar, 2 μm. Lower left, 1 μm. Upper right, 5 μm. PP, proplatelet; DMS, demarcation membrane system; BMC, bone marrow cell; black arrows indicate cytoplasmic fragmentation. (b) Confocal images of immunostained BM. Scale bars , 50 μm (in the left panel). Scale bars, 15 μm (in the right panel). MKs, proplatelets and platelets are shown by GPIb staining in green colour. Endoglin staining (red) labels vessels. DAPI, blue. (c) Intravital two-photon microscopy of BM MKs in the skull. Arrow shows (normal) proplatelet formation into BM sinusoids; dashed arrow indicates pre-released platelets within the BM. Scale bars, 25 μm. (d) BM MK spread on collagen I surface. White arrow indicates podosome formation in control MK. Scale bar, 15 μm. Images are representative of at least six versus six individuals. Full size image Figure 3: Premature platelet release into BM compartment. ( a ) TEM analysis of BM MKs (upper left: control MK). Scale bar, 2 μm. Lower left, 1 μm. Upper right, 5 μm. PP, proplatelet; DMS, demarcation membrane system; BMC, bone marrow cell; black arrows indicate cytoplasmic fragmentation. ( b ) Confocal images of immunostained BM. Scale bars , 50 μm (in the left panel). Scale bars, 15 μm (in the right panel). MKs, proplatelets and platelets are shown by GPIb staining in green colour. Endoglin staining (red) labels vessels. DAPI, blue. ( c ) Intravital two-photon microscopy of BM MKs in the skull. Arrow shows (normal) proplatelet formation into BM sinusoids; dashed arrow indicates pre-released platelets within the BM. Scale bars, 25 μm. ( d ) BM MK spread on collagen I surface. White arrow indicates podosome formation in control MK. Scale bar, 15 μm. Images are representative of at least six versus six individuals. Full size image Cytoskeletal alterations in Pfn1 −/− platelets To assess this in more detail, we analysed the cytoskeletal organization of circulating Pfn1 −/− platelets. Rapid-freezing electron microscopic analysis of Pfn1 −/− platelets revealed that their actin scaffold was partially disrupted ( Fig. 4a ; actin cytoskeleton of Pfn1 +/+ platelets ( n =102): 98% intact, 2% partially disrupted; actin cytoskeleton of Pfn1 −/− platelets ( n =116): 7.7% intact, 75.9% partially disrupted, 16.4% completely disrupted). As Pfn1 has been described as an important regulator of the actin cytoskeleton [10] , we determined actin levels and assembly in platelets. Total actin content in count-adjusted platelets was reduced ( Supplementary Fig. 6a ) and this was also evident by a reduced F-actin content per platelet ( Supplementary Fig. 6b ). Unexpectedly, actin assembly after platelet activation with different agonists was only slightly decreased in Pfn1 −/− platelets ( Supplementary Fig. 6c ). In contrast, other actin-regulatory proteins have been shown to have a more pronounced effect on F-actin assembly [19] . Surprisingly, the total tubulin content was increased in Pfn1 −/− MKs ( Supplementary Fig. 1c ) and platelets ( Supplementary Fig. 6a ). This also became evident by a higher number of microtubule coils, organized into a characteristic ring structure, designated as the marginal band ( Fig. 4a,b and Supplementary Fig. 6d ). Furthermore, the marginal band often seemed to have an altered morphology in mutant platelets, most frequently twisted into a figure of eight ( Fig. 4c ). We quantified platelets with twisted microtubules by analysing resting platelets on poly- L -lysine stained for α-tubulin. The majority of Pfn1 −/− platelets (55.7%; n =582) contained bent or twisted microtubules, whereas only 2.7% of control platelets ( n =1,037) showed an aberrant morphology of microtubules ( Supplementary Fig. 12c ). 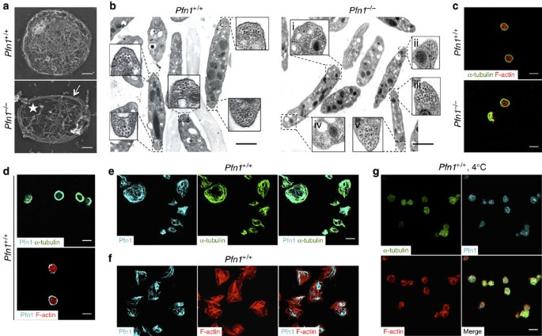Figure 4: Pfn1 co-localizes with microtubules and Pfn1 deficiency causes altered microtubule structure. (a) Visualization of the cytoskeleton of resting platelets on poly-L-lysine. Scale bar, 0.5 μm. Asterisk indicates disrupted actin scaffold. Arrow indicates thickened microtubule ring (marginal band). (b) TEM analysis of resting control andPfn1−/−platelets. Scale bar, 1 μm.i,iiandivshow altered microtubule distribution as revealed by not perpendicular but diagonally cut microtubules.iiiandvillustrate mutant platelets with abnormal high numbers of microtubule coils. (c) Confocal images of resting platelets. (d) Pfn1 localization in resting platelets and (e,f) spread platelets after 15 min on fibrinogen and (g) after cold-storage for 3.5 h. (c–g) Scale bars, 3 μm. Images are representative of at least five versus five individuals. Figure 4: Pfn1 co-localizes with microtubules and Pfn1 deficiency causes altered microtubule structure. ( a ) Visualization of the cytoskeleton of resting platelets on poly- L -lysine. Scale bar, 0.5 μm. Asterisk indicates disrupted actin scaffold. Arrow indicates thickened microtubule ring (marginal band). ( b ) TEM analysis of resting control and Pfn1 −/− platelets. Scale bar, 1 μm. i , ii and iv show altered microtubule distribution as revealed by not perpendicular but diagonally cut microtubules. iii and v illustrate mutant platelets with abnormal high numbers of microtubule coils. ( c ) Confocal images of resting platelets. ( d ) Pfn1 localization in resting platelets and ( e , f ) spread platelets after 15 min on fibrinogen and ( g ) after cold-storage for 3.5 h. ( c – g ) Scale bars, 3 μm. Images are representative of at least five versus five individuals. Full size image We next investigated the localization of Pfn1 in MKs and platelets. Pfn1 was strongly expressed in the MK body and proplatelets ( Supplementary Fig. 7a ), whereas a ring-shaped expression close to the membrane was observed in resting platelets, which was reminiscent of the platelet marginal band ( Fig. 4d ). A weak Pfn1 localization was found in the platelet cytoplasm, generally in small foci. In human platelets from healthy donors, a similar Pfn1 localization was seen ( Supplementary Fig. 7b ). After spreading of mouse platelets on fibrinogen, Pfn1 was redistributed in the cells but still strongly co-localized with α-tubulin ( Fig. 4e ) and was present in zones devoid of F-actin ( Fig. 4f ). Next, we tested whether Pfn1 is redistributed in control platelets upon cold-induced depolymerization of microtubules. After incubation of platelets at 4 °C, microtubules were completely disassembled and Pfn1 was re-localized to the cytoplasm, indicating that the localization of Pfn1 might be microtubule dependent ( Fig. 4g ). Increased stability of microtubules in Pfn1 −/− platelets To further investigate the organization and rearrangement of microtubules in Pfn1 −/− platelets, we performed spreading experiments on different matrices. Mutant platelets showed a delayed and aberrant spreading on fibrinogen, with a reduced F-actin content ( Fig. 5a , dashed arrows in lower panel) and disorganized microtubules that were randomly dispersed or twisted and failed to constrict into the cell centre ( Fig. 5a , arrow in lower panel). Similar to fibrinogen-coated surfaces (only 0.8±0.4% of Pfn1 −/− versus 20.7±0.3% of control platelets formed filopodia at 15-min time point; Supplementary Videos 3 and 4 ), Pfn1 −/− platelets could not form filopodia on a von Willebrand factor matrix (only 0.7±0.5% of Pfn1 −/− versus 60.0±3.6% of control platelets had formed filopodia at the 15-min time point) and maintained their thick marginal band ( Fig. 5b , arrows in lower panel), even after colchicine treatment ( Supplementary Fig. 8 ). Likewise, on a surface coated with collagen-related peptide (CRP) spread platelets could not reorganize their microtubule coils ( Supplementary Fig. 9 , arrow in lower panel). To our knowledge, this is the first evidence that Pfn1 is crucial for filopodia formation in platelets. 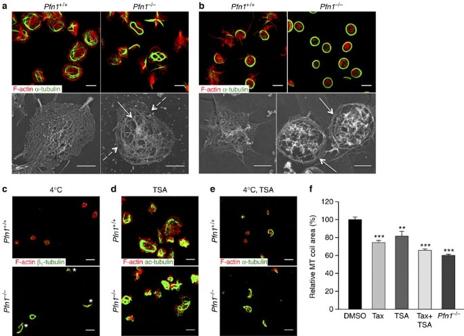Figure 5: Altered microtubule organization and increased stability contribute to microthrombocytopenia inPfn1−/−mice. Control andPfn1−/−platelets spread (15 min) on (a) fibrinogen- or (b) von Willebrand factor-coated surfaces were stained for F-actin (red) and α-tubulin (green), and analysed by confocal microscopy (upper panels) or processed for rapid-freezing electron microscopic analysis of the cytoskeleton (lower panels). Dashed arrows inahighlight the defective cortical F-actin meshwork and the arrow indicates disorganized microtubules in spreadPfn1−/−platelets. Arrows inbdenote thickened peripheral microtubule coils in Pfn1-deficient platelets. (c) Control andPfn1−/−platelets were incubated for 3.5 h at 4 °C, fixed on PLL-coated slides and stained for F-actin (red) and β1-tubulin (green). TSA-treated platelets (200 ng ml−1, 30 min) were allowed to (d) spread on a fibrinogen matrix or were (e) subjected to cold-induced microtubule disassembly assay, and subsequently stained for the indicated proteins. Scale bars, 3 μm (in confocal images) and 1 μm (in TEM images). (f) Platelets were treated with 10 μM taxol and/or 200 ng ml−1TSA for 30 min, fixed on PLL-coated slides and the relative platelet area was quantified using the microtubule coil as a measure. Values are mean±s.d. (n=5 versus 5). Images are representative of at least five versus five individuals. Unpaired Student’st-test: **P<0.01; ***P<0.001. Figure 5: Altered microtubule organization and increased stability contribute to microthrombocytopenia in Pfn1 −/− mice. Control and Pfn1 −/− platelets spread (15 min) on ( a ) fibrinogen- or ( b ) von Willebrand factor-coated surfaces were stained for F-actin (red) and α-tubulin (green), and analysed by confocal microscopy (upper panels) or processed for rapid-freezing electron microscopic analysis of the cytoskeleton (lower panels). Dashed arrows in a highlight the defective cortical F-actin meshwork and the arrow indicates disorganized microtubules in spread Pfn1 −/− platelets. Arrows in b denote thickened peripheral microtubule coils in Pfn1-deficient platelets. ( c ) Control and Pfn1 −/− platelets were incubated for 3.5 h at 4 °C, fixed on PLL-coated slides and stained for F-actin (red) and β 1 -tubulin (green). TSA-treated platelets (200 ng ml −1 , 30 min) were allowed to ( d ) spread on a fibrinogen matrix or were ( e ) subjected to cold-induced microtubule disassembly assay, and subsequently stained for the indicated proteins. Scale bars, 3 μm (in confocal images) and 1 μm (in TEM images). ( f ) Platelets were treated with 10 μM taxol and/or 200 ng ml −1 TSA for 30 min, fixed on PLL-coated slides and the relative platelet area was quantified using the microtubule coil as a measure. Values are mean±s.d. ( n =5 versus 5). Images are representative of at least five versus five individuals. Unpaired Student’s t -test: ** P <0.01; *** P <0.001. Full size image Microtubules in Pfn1 −/− platelets were highly acetylated ( Supplementary Fig. 10a–d ) and could withstand disassembly after incubation at 4 °C ( Fig. 5c ) or treatment with the microtubule-destabilizing toxin, colchicine ( Supplementary Fig. 11a ), suggesting an increased microtubule stability. Therefore, we tested whether toxin-induced stabilization of microtubules could mimic the tubulin phenotype observed in Pfn1 −/− platelets. Treatment with the microtubule-stabilizing toxin taxol resulted in a moderate increase of radially organized microtubules in control platelets, while spread Pfn1 −/− platelets maintained the circular or twisted microtubules ( Supplementary Fig. 11b ). Thus, taxol alone is not sufficient to reproduce the microtubular alterations of spread Pfn1 −/− platelets. In contrast, preincubation with the histone-deacetylase inhibitor trichostatin A (TSA) could partially mimic the Pfn1 −/− microtubule phenotype by preserving hyperacetylated and disorganized microtubules in spread control platelets and increasing microtubule acetylation in Pfn1 −/− platelets ( Fig. 5d ). These highly acetylated microtubules in control and Pfn1 −/− platelets were also less prone to cold-induced disassembly ( Fig. 5e ). Furthermore, isolation of the tubulin cytoskeleton after treatment with colchicine or the histone deacetylase inhibitor TSA via ultracentrifugation was performed and the different fractions were tested for tubulin and acetylated tubulin sedimentation. These results revealed an increased amount of sedimented ( Fig. 6a ) and acetylated ( Fig. 6b ) tubulin in the insoluble fraction after colchicine treatment in samples of Pfn1 −/− platelets, supporting the microscopic findings that microtubules cannot be rearranged in mutant platelets. Hence, we conclude that hyperacetylated, stiff microtubules might cause the aberrant microtubule organization in Pfn1 −/− platelets. In addition, the altered microtubule stability and organization appears to be independent of the actin cytoskeletal defects as control platelets pre-incubated with latrunculin A disassembled their microtubules on cold storage at 4 °C ( Supplementary Fig. 11c ). Next, we examined whether the increased microtubule stability could account for the reduced size of Pfn1 −/− platelets. Determination of the area delimited by the marginal band in control platelets showed a decrease in platelet size after treatment with taxol (74.41±2.33% compared with dimethyl sulphoxide control 100%), TSA (81.53±5.44%), or the combination of both (65.62±1.59%; untreated Pfn1 −/− platelets 60.8% of control, Fig. 5f and Supplementary Fig. 12a ). Measurement of the filamentous actin content in toxin-treated resting platelets showed that the toxins did not interfere with the actin cytoskeleton ( Supplementary Fig. 12b ). These results suggested that increased microtubule stability might contribute to the smaller size of Pfn1 −/− platelets. Of note, it has been recently shown that antagonistic microtubule motor proteins maintain the platelet marginal band under resting conditions, and that functional changes can lead to microtubule coiling accompanied by platelet shape change [20] . Therefore, it is tempting to speculate that the small Pfn1 −/− platelets might exhibit an imbalanced microtubule motor protein function, consequently leading to twisted or bent microtubules. However, further studies are required to test this hypothesis. 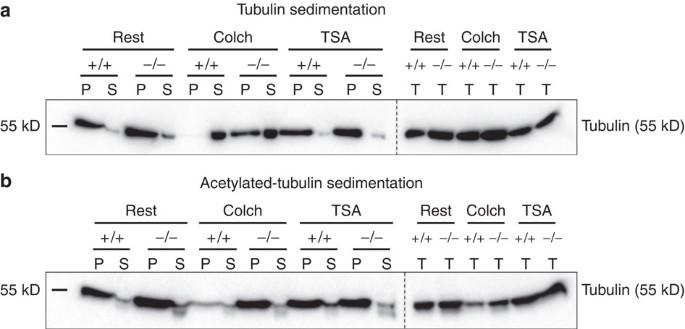Figure 6: Increased microtubule (MT) stability inPfn1−/−platelets. Tubulin cytoskeleton was isolated via ultracentrifugation and immunoblotted against (a) tubulin or (b) acetylated tubulin. Insoluble fraction (pellet, P); soluble fraction (supernatant, S); rest, resting; colch, 10 μM colchicine; TSA, 200 ng ml−1TSA, deacetylase inhibitor; T, total protein. Figure 6: Increased microtubule (MT) stability in Pfn1 −/− platelets. Tubulin cytoskeleton was isolated via ultracentrifugation and immunoblotted against ( a ) tubulin or ( b ) acetylated tubulin. Insoluble fraction (pellet, P); soluble fraction (supernatant, S); rest, resting; colch, 10 μM colchicine; TSA, 200 ng ml −1 TSA, deacetylase inhibitor; T, total protein. Full size image Altered microtubule rearrangement in WAS patients’ platelets Pfn1 −/− mice are the first animal model displaying a microthrombocytopenia and thus represent a unique system to study the molecular causes and (patho-) physiological consequences of this haematopoietic defect. In humans, microthrombocytopenia is the central hallmark of the WAS [2] , which was interestingly not reproduced in WASp-deficient mice that have normal-sized platelets [6] , [16] . Although, our analysis of Wasp −/− mouse platelets revealed an increased content of tubulin similar to Pfn1 −/− platelets ( Supplementary Figs 1c and 13b ), microtubule stability or reorganization during spreading or cold-induced microtubule disassembly was not affected in these cells ( Supplementary Fig. 13c,d ). To assess whether an increased microtubule stability may contribute to microthrombocytopenia in humans, we analysed blood samples of four WAS patients. Patient 1 was a 2-year-old male carrying a c.290C>T p.Arg86Cys mutation in the WAS gene. At the day of consultation, the patient had a platelet count of 11 × 10 3 μl −1 and the mean platelet volume could not be determined with an automated blood cell analyser (Sysmex), presumably due to an aberrant platelet morphology and size. Patient 2 was a 7-year-old male with a c.336T>G p.Leu101Arg mutation in the WAS gene. During the first year of his life he suffered from severe brain haemorrhage due to low numbers of circulating platelets, which was the reason for subsequent therapeutic splenectomy. At the day of consultation, he presented with a platelet count of 128 × 10 3 μl −1 and a mean platelet volume of 7.5 fl as determined by a Sysmex analyser. In contrast to patient 1 and 2, patient 3 (male, 5-month-old, c.559+1G>A splice-site mutation in intron 6 of the WAS gene) suffered from eczema, petechiae, lymphocytopenia, recurrent infections and anisocytosis, and required platelet transfusions due to low platelet numbers (32 × 10 3 μl −1 at the day of consultation). Patient 4 was an 18-year-old male with a frameshift mutation in exon 10 (c.1075delC p.Pro360His fsX85) of the WAS gene and had a history of recurrent infections and arthritis. At the day of consultation, he presented with a platelet count of 29 × 10 3 μl −1 . The analysis of the cytoskeletal organization of WAS patients’ platelets revealed an increased content and highly altered organization of the microtubules ( Fig. 7a and Supplementary Fig. 14a ). Three major microtubule organization types could be distinguished: (I) platelets with a normally organized but thickened marginal band, (II) platelets that contained microtubules in the platelet centre ( Fig. 7a , Supplementary Fig. 14a , arrows, and Supplementary Videos 6, 8, 10 and 12 ) and (III) platelets with twisted and disorganized microtubules ( Fig. 7a , Supplementary Fig. 14a , dashed arrows, and Supplementary Videos 7, 9, 11 and 13 ). Although platelets of healthy controls ( Supplementary Video 5 ) displayed a discoid shape, the platelets of patient 1 ( Supplementary Videos 6 and 7 ), 2 ( Supplementary Videos 8 and 9 ), 3 ( Supplementary Videos 10 and 11 ) and 4 ( Supplementary Videos 12 and 13 ) were often curved in shape, most probably attributed to misarranged microtubules. Next, control and WAS patients’ platelets were challenged with colchicine ( Fig. 7b and Supplementary Fig. 14b ) or chilled at 4 °C ( Fig. 7c and Supplementary Fig. 14c ). Contrary to control samples, under both tested conditions microtubules of WAS patients’ platelets were still prominently visible, disorganized, bent or twisted ( Fig. 7b,c and Supplementary Fig. 14b,c ), and highly acetylated ( Fig. 7d and Supplementary Fig. 14d ). Similar to Pfn1 −/− platelets, electron microscopic analyses of platelets from patient 2 and 3 showed an increased number of microtubules (10.58±2.04 in controls versus 14.86±2.66 in patients) with an altered organization ( Fig. 7e and Supplementary Fig. 14e ). Even though the splenectomy of patient 2 resulted in increased platelet numbers, the microtubule cytoskeleton was still severely altered and disorganized. Of note, WASP heterozygosity in case of a female carrier moderately affected microtubule stability and organization ( Supplementary Fig. 14a–c,e ). Interestingly, Pfn1 was mislocalized in platelets of WAS patients 1, 3 and 4, suggesting that WASp and Pfn1 interact with each other in human platelets ( Fig. 8 ). Together, these data reveal that platelets from WAS patients display defective microtubule reorganization as observed in Pfn1 −/− platelets. 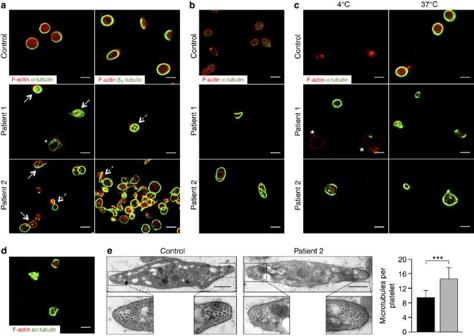Figure 7: Platelets of WAS patients resemble the microtubule phenotype ofPfn1−/−platelets. (a) Poly-L-lysine-immobilized resting platelets from two male WAS patients were stained for F-actin (red) and different tubulin isoforms (green), and analysed by confocal microscopy. Patient 1: 2 years, without therapeutic intervention, carrying a R86C mutation in exon 2 of theWASgene; Patient 2: 7 years, underwent therapeutic splenectomy in his first year of life, carrying a L101R mutation in exon 3 of theWASgene. Microtubules in WAS patients’ platelets were challenged with (b) colchicine (10 μM) or (c) by incubation at 4 °C for 3.5 h. (d) Resting platelets of patient 2 were stained for acetylated tubulin (green) and F-actin (red). (e) TEM images revealed an increased number and aberrant organization of the microtubules in the WAS patients’ platelets (grey bar) as compared with that of healthy controls (black bar). Values are mean±s.d. (n=71 versus 46 platelets). Scale bars, 3 μm (a–d) and 1 μm (e). Unpaired Student’st-test; ***P<0.001. Figure 7: Platelets of WAS patients resemble the microtubule phenotype of Pfn1 −/− platelets. ( a ) Poly- L -lysine-immobilized resting platelets from two male WAS patients were stained for F-actin (red) and different tubulin isoforms (green), and analysed by confocal microscopy. Patient 1: 2 years, without therapeutic intervention, carrying a R86C mutation in exon 2 of the WAS gene; Patient 2: 7 years, underwent therapeutic splenectomy in his first year of life, carrying a L101R mutation in exon 3 of the WAS gene. Microtubules in WAS patients’ platelets were challenged with ( b ) colchicine (10 μM) or ( c ) by incubation at 4 °C for 3.5 h. ( d ) Resting platelets of patient 2 were stained for acetylated tubulin (green) and F-actin (red). ( e ) TEM images revealed an increased number and aberrant organization of the microtubules in the WAS patients’ platelets (grey bar) as compared with that of healthy controls (black bar). Values are mean±s.d. ( n =71 versus 46 platelets). Scale bars, 3 μm ( a – d ) and 1 μm ( e ). Unpaired Student’s t -test; *** P <0.001. 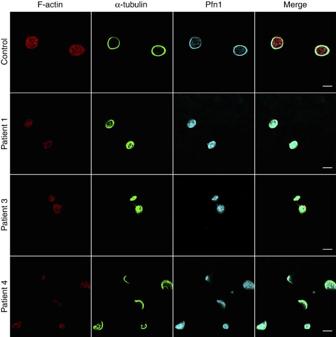Figure 8: Mislocalization of Pfn1 in platelets of WAS patients. Resting platelets of healthy human controls and WAS patients 1, 3 and 4 were immobilized on poly-L-lysine and stained for F-actin (red), α-tubulin (green) and Pfn1 (cyan). Scale bar, 3 μm. Full size image Figure 8: Mislocalization of Pfn1 in platelets of WAS patients. Resting platelets of healthy human controls and WAS patients 1, 3 and 4 were immobilized on poly- L -lysine and stained for F-actin (red), α-tubulin (green) and Pfn1 (cyan). Scale bar, 3 μm. Full size image Mutations in the WAS gene cause a complex syndrome, including microthrombocytopenia [2] , but the underlying molecular mechanisms have not been elucidated. Unexpectedly, Wasp −/− or WIP −/− mice do not completely reproduce the clinical symptoms described for WAS patients, particularly with respect to the severe microthrombocytopenia [2] , [7] , [16] , suggesting that WASp deficiency may not directly, but rather indirectly, affect platelet size determination through so far undefined mechanisms. We show that Pfn1 −/− mice do fully reproduce the MK/platelet phenotype found in WAS patients. In addition, our data establish Pfn1 as a new and highly relevant negative regulator of microtubule stability and reorganization. These findings indicate that the MK/platelet phenotype in WAS might be caused by altered Pfn1 function and/or localization ( Fig. 8 ). In support of this, we could show that comparable to Pfn1 −/− platelets, platelets of all three WAS patients contained severely misarranged and hyperstable microtubules that might represent the molecular cause of the reduced platelet size. To date, no Pfn1-null patients have been reported, most probably due to embryonic lethality as described for constitutive Pfn1-deficient mice [12] . Even though our studies indicate a co-localization of Pfn1 and platelet microtubule coils, we could not detect direct Pfn1 binding to microtubules ( Supplementary Fig. 15 ). However, we speculate that Pfn1 might be indirectly linked to microtubules by a protein complex consisting of one or more of its over 50 interaction partners ( Fig. 9 ) [11] . For example, Pfn1 might be indirectly linked to the microtubule cytoskeleton via its interaction with formins, which are well described to bind microtubules [21] . Moreover, it was reported that large amounts of tubulin were found in the Pfn1 complex, but direct Pfn1-tubulin binding was also not detected [22] . A possible hypothesis is that Pfn1 binds to phospholipids in the membrane and orchestrates microtubule stabilization/rearrangement within a multi-protein complex, possibly involving WASp and/or WIP ( Fig. 9 ). Even though Pfn1 was reported to interact with the ubiquitously expressed WASp homologue, N-WASp [14] , no direct interaction with haematopoietic WASp has been reported so far. Pfn1, however, is known to indirectly couple to WASp via WIP [15] , which we could also show by co-immunoprecipitation of Pfn1 and WASp ( Supplementary Fig. 16 ), thus further linking Pfn1 to WAS. Moreover, it has been suggested that Pfn1 might act as a direct activator of WASp or formins [11] . Consequently, the striking similarities between platelets of Pfn1 −/− mice and WAS patients, along with the close localization of Pfn1 to microtubules observed in T cells and, to a lower extent, in fibroblasts ( Supplementary Fig. 17 ), point to a potential involvement of Pfn1 in the pathogenesis of the WAS. Therefore, it will be interesting to investigate a possible contribution of Pfn1-mediated alteration of microtubule stability to the development of immunodeficiency in WAS patients. The differences between WAS patients and Wasp −/− mice (severity of thrombocytopenia, platelet size and microtubule reorganization) remain enigmatic. It was previously hypothesized that small platelets in WAS patients may escape splenic macrophages, and the lack of small platelets and the only moderate thrombocytopenia in Wasp −/− mice results from the smaller-sized mouse platelets as compared with human platelets. However, it has to be noted that in contrast to WAS patients we could not find altered platelet microtubule stability in WASp- ( Supplementary Fig. 13 ) or WIP-deficient mice ( Supplementary Fig. 18 ). A possible role of the WASp homologue N-WASp in these processes needs to be determined. Additional support for a possible involvement of Pfn1 in the pathogenesis of WAS is provided by the growing evidence that abnormal microtubule rearrangement contributes to the development of diseases, for example, as recently shown for Parkinson’s disease [23] , [24] . 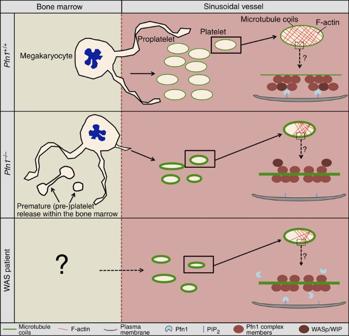Figure 9: Hypothetical model. Control BM MKs form proplatelets into the sinusoidal vessel where platelets are released from proplatelets. MT coils form a ‘ring-like’ structure designated as the marginal band. Pfn1 can bind to PIP2at the membrane and regulate via its interaction partners, including WASp/WIP, microtubule reorganization.Pfn1−/−mice display premature platelet release into the BM compartment.Pfn1−/−MKs produce less and smaller-sized platelets into the circulation, which have a thicker marginal band and a partially disrupted actin cytoskeleton. Lack of Pfn1 results in unrestrained function of Pfn1 interaction partners with consequent defective MT reorganization. Less is known about platelets derived from BM MKs of WAS patients. WAS patients display a microthombocytopenia as observed inPfn1−/−mice. Increased MT stability in platelets of WAS patients might be caused by altered localization and function of Pfn1 and Pfn1 interaction partners. Figure 9: Hypothetical model. Control BM MKs form proplatelets into the sinusoidal vessel where platelets are released from proplatelets. MT coils form a ‘ring-like’ structure designated as the marginal band. Pfn1 can bind to PIP 2 at the membrane and regulate via its interaction partners, including WASp/WIP, microtubule reorganization. Pfn1 −/− mice display premature platelet release into the BM compartment. Pfn1 −/− MKs produce less and smaller-sized platelets into the circulation, which have a thicker marginal band and a partially disrupted actin cytoskeleton. Lack of Pfn1 results in unrestrained function of Pfn1 interaction partners with consequent defective MT reorganization. Less is known about platelets derived from BM MKs of WAS patients. WAS patients display a microthombocytopenia as observed in Pfn1 −/− mice. Increased MT stability in platelets of WAS patients might be caused by altered localization and function of Pfn1 and Pfn1 interaction partners. Full size image In summary, we show that Pfn1 −/− mice display a microthrombocytopenia strongly resembling the platelet phenotype of WAS patients ( Table 1 ). In addition, we identified a central role for Pfn1 in preserving the integrity of the microtubule cytoskeleton. Similar to Pfn1 −/− platelets, we revealed altered microtubule rearrangement and organization in platelets of WAS patients. Based on our findings, we speculate that WASp acts as a modulator of Pfn1 function in MKs, and that this process is disturbed in WAS patients, leading to the known platelet formation defect. Table 1 Summary and comparison of major findings between Pfn1 −/− mice, WAS patients and WASp −/− mice. Full size table Mice Conditional Pfn1-deficient mice were generated by intercrossing Pfn1 fl/fl mice (exon 2 flanked by loxP sites) with mice carrying the Cre-recombinase under the platelet factor 4 ( Pf4 ) promoter [25] . Pfn1 fl/fl mice were obtained from EUCOMM (European Conditional Mouse Mutagenesis Program, Strain ID EM:03711) and Pf4-Cre mice were kindly provided by Dr Radek Skoda. All mice used in experiments were 12- to 16 weeks old and sex-matched, if not stated otherwise. For experiments on MKs, only male animals were used. All animal experiments were approved by the district government of Lower Frankonia (Bezirksregierung Unterfranken). WASp-null [6] and WIP-null [26] mice were maintained on a C57Bl/6 background. Approval for animal research was granted by the Harvard Medical Area Standing Committee, according to the National Institutes of Health standards and as outlined in the Institute for Laboratory Animal Research Guide for Care and Use of Laboratory Animals. Platelet preparation Mice were bled under isoflurane anaesthesia. Blood was collected in heparin (20 U ml −1 , Ratiopharm) and centrifuged twice for 6 min at 300 g . Platelet-rich plasma (PRP) was supplemented with 2 μl of apyrase (0.02 U ml −1 ; A6410, Sigma-Aldrich) and 5 μl PGI 2 (0.1 μg ml −1 ; P6188, Sigma-Aldrich), and platelets were pelleted by centrifugation for 5 min at 800 g , washed twice with Tyrodes–HEPES buffer (N-2-hydroxyethyl-piperazine-N′2-ethanesulphonic acid; 134 mM NaCl, 0.34 mM Na 2 HPO 4 , 2.9 mM KCl, 12 mM NaHCO 3 , 5 mM HEPES, 5 mM glucose, 0.35% BSA, pH 7.4) containing 2 μl apyrase and 5 μl PGI 2 . Blood was collected under protocols, including informed consent approved by the Ethics Committee of the University of Würzburg. Fresh blood samples of WAS patients and healthy volunteers were collected in 1/10 volume of acid–citrate–dextrose and centrifuged for 10 min at 200 g . PRP was collected, supplemented with 2 μl of apyrase (0.02 U ml −1 , Sigma-Aldrich) and 5 μl PGI 2 (0.1 μg ml −1 , Sigma-Aldrich) per ml PRP. Before adherence to poly-L-lysine-coated slides, platelets were pelleted by centrifugation for 10 min at 800 g and washed twice with Tyrodes–HEPES buffer containing 2 μl apyrase and 5 μl PGI 2 . The samples were allowed to rest for 30 min at 37 °C. Flow cytometry Diluted blood (1:20) was incubated for 15 min at room temperature (RT) with fluorophore-conjugated antibodies (2 μg ml −1 ) directed against platelet surface glycoproteins [19] . Platelet count, size (forward scatter) and glycoprotein expression were assessed using a FACSCalibur (BD Biosciences) flow cytometer. Blood smears Blood smears were generated by placing a 5-μl drop of venous blood at one end of a glass slide and pulling the blood drop longitudinally across the slide using a second glass slide at a 45° angle. Slides were allowed to dry, fixed with May-Grünwald’s solution (MG500, Sigma-Aldrich) and stained with Giemsa’s solution (GS500, Sigma-Aldrich) according to Pappenheim. Slides were analysed with an inverted Leica DMI 4000 B microscope. Co-immunoprecipitation Washed resting or CRP-treated platelets were lysed by sonification under low-salt conditions in PIPES (piperazine- N , N -bis-2-ethanesulphonic acid; pH 7.0) buffer, supplemented with protease inhibitors (PI; P8340, Sigma-Aldrich) and phenylmethylsulphonylfluorid (#8553, Cell Signaling). Platelet lysates were precleared by incubation with protein A-sepharose (17-0780-01, GE Healthcare) for 1 h at 4 °C under agitation. WASp was precipitated by incubation of the cleared lysates with a mouse anti-WASp antibody (3 μg, sc-13139 (B-9), Santa Cruz Biotechnology Inc.)-coated protein A-sepharose overnight at 4 °C. Supernatant (SN) was collected and the sepharose pellet was washed extensively with PIPES buffer supplemented with PI before 2 × Laemmli buffer was added. Samples (total lysate, immunoprecipitation (IP) and SN) were separated by SDS–PAGE and immunoblotted with a rabbit anti-Pfn1 (1 μg ml −1 , P7749, Sigma-Aldrich, polyclonal) or a rabbit anti-WASp (1 μg ml −1 , #4860, Cell Signaling) antibody. Immunoblotting Denatured platelet or MK lysates were separated by SDS–PAGE and blotted onto polyvinylidene difluoride membranes. Pfn1 (1 μg ml −1 , P7749, Sigma-Aldrich), β-actin (1 μg ml −1 , #4970, Cell Signaling) or tubulin (0.5 μg ml −1 , MAB1864 (YL1/2), Millipore) were probed with the respective antibodies and detected using horseradish peroxidase-conjugated secondary antibodies (0.33 μg ml −1 ) and enhanced chemiluminescence solution (JM-K820-500, MoBiTec). Images were recorded using a MultiImage II FC Light Cabinet (Alpha Innotech Corperation) device. As loading control, GPIIIa or β-actin levels were determined. Uncropped immunoblotting images are shown in Supplementary Figs 19 and 20 . Microtubule sedimentation Resting or toxin-treated (10 μM colchicine (A4082, AppliChem); 200 ng ml −1 , TSA (A7812, AppliChem)) platelets (5.7 × 10 7 ) were lysed in PHEM buffer containing 1% Triton X-100, 6 μM taxol (A4667, AppliChem) and PIs (P8340, Sigma-Aldrich). Polymerized and soluble fractions were separated by centrifugation for 30 min at 100,000 g and 37 °C in a TLA-100 rotor (Beckman Coulter). Total platelet lysates, soluble SNs and insoluble pellets (P) were supplemented with SDS–PAGE buffer containing 5% β-mercaptoethanol (M6250, Sigma-Aldrich). Samples were separated by SDS–PAGE, blotted onto polyvinylidene difluoride membranes and probed with anti-tubulin (0.5 μg ml −1 , MAB1864 (YL1/2), Millipore) and anti-acetylated tubulin (1 μg ml −1 , sc-23950 (6-11B-1), Santa Cruz Biotechnology Inc.) antibodies. Semi-quantitative reverse transcription–PCR Total platelet RNA was isolated after lysis using TRIzol reagent (15596018, Invitrogen) and tissue RNA was gained using the Qiagen RNeasy kit. To generate complementary DNA, 1 μg RNA was reverse transcribed with the SuperScript II reverse transcriptase (18064014, Invitrogen) according to the manufacturer’s instructions. Amplification of Pfn isoforms was performed with the respective primer pairs: Pfn1_RT_forw: 5′-GCCATCGTAGGCTACAAGGACTCG-3′ and Pfn1_RT_rev: 5′-CCACCGTGGACACCTTCTTTGC-3′, expected product size 305 bp for control and 113 bp for Pfn1 knockout; Pfn2_RT_forw: 5′-GCTACGTGGATAACCTGATGTGCG-3′ and Pfn2_RT_rev: 5′-CCCCTAATACTTAACAGTCTGCCTAGC-3′, expected product size 436 bp; Pfn3_RT_forw: 5′-GCAAGCACAAGTTGCTGGGACTG-3′ and Pfn3_RT_rev: 5′-GACCCGTCTGCAGAAAGGTGTGC-3′, expected product size 224 bp; Pfn4_RT_forw: 5′-GCTGGGGACGAAACACGTGG-3′ and Pfn4_RT_rev: 5′-CTTCTCTGTGGCTTCCACGCAGAC-3′, expected product size 322 bp. GAPDH transcripts were determined as control with the primer pair GAPDH_RT_forw: 5′-GCAAAGTGGAGATTGTTGCCAT-3′ and 5′-CTTGACTGTGCCGTTGAATTT-3′, and an expected product size of 108 bp. Determination of platelet life span The clearance of platelets from the circulation was determined by the retro-orbital injection of 5 μg DyLight 488-labelled anti-GPIX antibody in PBS into male mice. The percentage of labelled platelets was determined by daily blood withdrawal and subsequent analysis by flow cytometry using fluorophore-conjugated platelet-specific antibodies. Splenectomy Platelet count and size of female and male mice was determined by flow cytometry before surgical splenectomy. The surgical site on anaesthetized mice was sterilely prepared and a 1-cm paramedian incision over the left upper quadrant was made. After the spleen was identified, blood supply was stopped by ligation of vascular pedicles with surgical suture material and the spleen was removed. Mice were monitored for 48 h for signs of internal bleeding and infection. After a recovery period of 6 days, platelet counts and size were followed over time by flow cytometry. Macrophage depletion Anaesthetized female and male mice were retro-orbitally injected with clodronate-encapsulated or PBS-encapsulated liposomes (2 μl per g body weight). Blood was taken at 0, 24, 48, 72 and 96 h after injection and, subsequently, platelet counts and size were determined by flow cytometry. Platelet spreading on fibrinogen, CRP or vWF Coverslips were either coated with fibrinogen (100 μg ml −1 ; F4883, Sigma-Aldrich), CRP [27] (6 μg ml −1 ) or rabbit anti-human-vWF antibody (0.25 μg ml −1 , A0082, DAKO) overnight at 4 °C. For spreading on fibrinogen, platelets were stimulated with 0.01 U ml −1 thrombin (10602400001, Roche) and allowed to spread for the indicated time points. For spreading on vWF, the anti-human-vWF antibody-coated slides were incubated with mouse plasma to allow vWF binding, and platelets were pre-incubated with 40 μg ml −1 eptifibatide (Millenium Pharmaceuticals) and co-stimulated with 1 U ml −1 botrocetin (Pentapharm Ltd). If indicated, platelets were pre-incubated with toxins interfering with cytoskeletal dynamics such as colchicine (10 μM; A4082, AppliChem), taxol (10 μM; A4667, AppliChem) or latrunculin A (2.5 μM; sc-202691, Santa Cruz Biotechnology Inc.) before spreading assay. After the indicated time points, platelets were either fixed with 4% paraformaldehyde (PFA) in PBS and analysed or processed for immunofluorescence staining of the cytoskeleton. Therefore, platelets were fixed and permeabilized in PHEM buffer (60 mM PIPES, 25 mM HEPES, 10 mM ethylene glycol tetraacetic acid, 2 mM MgCl 2 , pH 6.9) supplemented with 4% PFA and 1% IGEPAL CA-630, stained with anti-α-tubulin Alexa F488 (3.33 μg ml −1 , 322588 (B-5-1-2), Invitrogen), anti-β 1 -tubulin (2.5 μg ml −1 , T4026 (TUB 2.1), Sigma-Aldrich), anti-acetyl-tubulin (2 μg ml −1 , sc-23950 (6-11B-1), Santa Cruz Biotechnology Inc.), anti-Pfn1 (10 μg ml −1 , P7749, polyclonal, Sigma-Aldrich, directed against amino terminus; N-terminal antibody from Sigma-Aldrich was used in all experiments). Localization of Pfn1 in platelets was confirmed with a second anti-Pfn1 antibody directed against the carboxy terminus of Pfn1 (10 μg ml −1 , P7624, polyclonal), Sigma-Aldrich) or phalloidin-Atto647N (170 nM, 65,906, Fluka) and mounted with Fluoroshield (F6182, Sigma-Aldrich). All used fluorophore-conjugated secondary antibodies were purchased from Invitrogen. Samples were visualized using a Leica TCS SP5 confocal microscope (Leica Microsystems). Cold-induced microtubule disassembly Microtubules were depolymerized by incubation of platelets at 4 °C; reassembly was allowed by subsequent rewarming at 37 °C. Samples maintained at 4 °C and 37 °C, as well as rewarmed platelets were fixed and permeabilized in PHEM buffer supplemented with 4% PFA and 1% IGEPAL CA-630, and allowed to adhere to a poly- L -lysine-coated coverslips. Samples were immunostained using an anti-β 1 -tubulin (2.5 μg ml −1 , T4026, clone TUB 2.1, Sigma-Aldrich) or anti-α-tubulin Alexa F488 antibody (3.33 μg ml −1 , 322588 (B-5-1-2), Invitrogen) and visualized using a Leica TCS SP5 confocal microscope (Leica Microsystems). Transmission electron microscopy of platelets To analyse platelet ultrastructure, washed platelets were fixed with 2.5% glutaraldehyde (16210, Electron Microscopy Sciences) in 50 mM cacodylate buffer (12,201, pH 7.2; AppliChem). After embedding in epon 812 (14900, Electron Microscopy Sciences), ultra-thin sections were generated and stained with 2% uranyl acetate (22400, Electron Microscopy Sciences) and lead citrate (17,800, Electron Microscopy Sciences). Samples were visualized with an EM900 TEM (Carl Zeiss). Visualization of the platelet cytoskeleton using TEM The cytoskeleton of resting and spread platelets (15 min either on vWF, fibrinogen or CRP) was visualized by TEM. To prepare samples of resting platelets, washed platelets were spun (5 min at 280 g ) onto poly- L -lysine-coated (P8920, Sigma-Aldrich) coverslips in PHEM buffer supplemented with 0.75% Triton X-100 (X100, Sigma-Aldrich), 1 μM phalloidin (A1488, AppliChem), 1 μM taxol (A4667, AppliChem) and 0.1% glutaraldehyde. After washing with PHEM buffer containing 0.1 μM phalloidin and taxol, adherent platelets were fixed for 10 min in PHEM buffer supplemented with 1% glutaraldehyde. To prepare samples of spread platelets, washed platelets were spun (5 min at 280 g ) onto fibrinogen- (100 μg ml −1 , F4883, Sigma-Aldrich), CRP- or plasma vWF-coated slides in Tyrodes–HEPES buffer (134 mM NaCl, 0.34 mM Na 2 HPO 4 , 2.9 mM KCl, 12 mM NaHCO 3 , 5 mM HEPES, 1 mM CaCl 2 , 5 mM glucose, 0.35% BSA, pH 7.4), stimulated with 0.01 U ml −1 thrombin (10602400001, Roche) or 1 U ml −1 botrocetin, and incubated for 15 min. To stop the reaction, coverslips were incubated for 5 min with PHEM buffer containing 0.75% Triton X-100, 0.1% glutaraldehyde, 1 μM phalloidin and taxol. After a quick washing step with PHEM buffer containing 0.1 μM phalloidin and taxol, adherent platelets were fixed for 10 min in PHEM buffer supplemented with 1% glutaraldehyde. Coverslips were extensively washed in ultra-pure water, rapidly frozen in a liquid helium-cooled copper block, transferred to a liquid nitrogen-cooled stage, freeze-dried at −90 °C and metal cast with 1.2 nm of tantalum-tungsten with rotation at 45° and 3 nm of carbon at 90° without rotation. Replicas were floated, picked up on formvar-carbon-coated grids and examined in a JEOL 1200-EX TEM at 80 kV. Actin polymerization Washed platelets were incubated with a Dylight-649-labelled anti-GPIX antibody derivative (20 μg ml −1 ). Subsequently, platelets were either left unstimulated or were stimulated with the indicated agonists for 2 min. Platelets were fixed with 0.55 volume of 10% PFA in PHEM buffer and treated with 0.1 volume 1% Triton X-100. Subsequently, the platelets were stained with 10 μM phalloidin-fluorescein isothiocyanate (P5282, Sigma-Aldrich) for 30 min and analysed on a FACSCalibur. Histology Three-micrometre-thick sections of formalin-fixed paraffin-embedded spleens and femora of male mice were prepared, deparaffinized and stained with haematoxylin (MHS32, Sigma-Aldrich) and eosin (318906, Sigma-Aldrich). MK number, morphology and localization were analysed with an inverted Leica DMI 4,000 B microscope. Immunofluorescence staining on whole femora cryosections Femora of male mice were isolated, fixed with 4% PFA (A3813, AppliChem) and 5 mM sucrose (S0389, Sigma-Aldrich), transferred into 10% sucrose in PBS and dehydrated using a graded sucrose series. Subsequently, the samples were embedded in Cryo-Gel (39475237, Leica Biosystems) and shock frozen in liquid nitrogen. Frozen samples were stored at −80 °C. Seven-micrometre-thick cryosections were generated using the CryoJane tape transfer system (Leica Biosystems) and probed with Alexa488-conjugated anti-GPIb [28] antibodies (7A9, 1.33 μg ml −1 ), to specifically label platelets and MKs, and Alexa647-conjugated anti-CD105 antibodies (3.33 μg ml −1 , 120402 (MJ7/18), Biolegend) to stain the endothelium. Nuclei were stained using DAPI (4′,6-diamidino-2-phenylindole; 1 μg ml −1 , D1306, Invitrogen). Samples were visualized with a Leica TCS SP5 confocal microscope (Leica Microsystems). Two-photon intravital microscopy of the BM Male and female mice were anaesthetized and a 1-cm incision was made along the midline to expose the frontoparietal skull, while carefully avoiding damage to the bone tissue. The mouse was placed on a customized metal stage equipped with a stereotactic holder to immobilize its head [29] . BM vasculature was visualized by injection of tetramethylrhodamine dextran (8 μg per g body weight, 2 MDa, Molecular Probes). Platelets and MKs were antibody stained (0.6 μg per gram body weight anti-GPIX-Alexa Fluor 488). Images were acquired with a fluorescence microscope equipped with a × 20 water objective with a numerical aperture of 0.95 and a TriM Scope II multiphoton system (LaVision BioTec), controlled by ImSpector Pro-V380 software (LaVision BioTec). Emission was detected with HQ535/50-nm and ET605/70-nm filters. A tunable broad-band Ti:Sa laser (Chameleon, Coherent) was used at 760 nm to capture Alexa Fluor 488 and rhodamine dextran fluorescence. ImageJ software (NIH) was used to generate movies. TEM of bone marrow megakaryocytes For TEM of MKs, BM was flushed from 12- to 16-week-old male mice using Karnovsky fixative (2% PFA, 2.5% glutaraldehyde in 0.1 M cacodylate buffer) and incubated overnight at 4 °C. Subsequently, fatty components of the samples were fixed with 2% osmium tetroxide in 50 mM sodium cacodylate (pH 7.2), stained with 0.5% aqueous uranyl acetate, dehydrated with a graded ethanol series and embedded in Epon 812. Ultra-thin sections were stained with 2% uranyl acetate (in 100% ethanol) followed by lead citrate. Images were taken on a Zeiss EM900 TEM (Zeiss). Plasma TPO levels Plasma TPO levels were determined using a Mouse Thrombopoietin Quantikine ELISA Kit (DY488, R&D Systems). Briefly, plasma was collected, diluted (1:5 in Reagent Diluent) and immediately applied as duplicates onto the anti-TPO-IgG coated 96-well plate and incubated for 2 h at RT. The plate was washed five times and incubated for 2 h with 100 μl of horseradish peroxidase-conjugated anti-mouse TPO antibodies. After another five washing steps, tetramethylbenzidine solution was added and incubated for 30 min at RT. The reaction was aborted by the addition of 100 μl of diluted hydrochloric acid. Optical densities of the samples were determined using a Multiskan Ascent (96/384) plate reader (MTX Lab Systems) at 450 nm. Wavelength correction was performed at 570 nm. In vitro differentiation of fetal liver cell-derived MKs The livers of 13.5-to 14.5-day-old female and male mouse embryos were isolated from time-mated female mice and a single cell suspension was prepared in MK medium (IMDM medium containing 10% FCS, 1% penicillin/streptomycin (31980097, Gibco) and 50 ng ml −1 recombinant TPO [30] ). The homogenized liver cells were cultured for 72 h at 37 °C and 5% CO 2 , and mature MKs were enriched on day 3 of culturing using a BSA density gradient (3% and 1.5% BSA in PBS; A7030, Sigma-Aldrich). On day 4, the percentage of proplatelet-forming MKs was determined by counting the total number of MKs as well as the number of proplatelet-forming MKs under a light microscope (Zeiss). In vitro differentiation and cultivation of BM MKs Haematopoietic stem cells were isolated from male mouse BM single cell suspensions using a magnetic bead-based negative depletion kit (anti-rat-IgG Dynabeads, Invitrogen) in combination with rat-anti-mouse antibodies directed against CD45R/B220, TER-119, CD3, Ly-6G/C and CD11b (each 0.5 μg per 10 7 cells, 103,216 (RA3-6B2), 116,214 (TER-119), 100,208 (17A2), 108,414 (RB6-8C5), 101,214 (M1/70), Biolegend). Experiments were performed according to the manufacturer’s protocol. Cells were cultured in MK medium supplemented with 50 μg ml −1 recombinant hirudin (Schering) at 37 °C, 5% CO 2 for 3 days, before MK enrichment using a two-step BSA density gradient. On day 4, the percentage of proplatelet-forming MKs was determined using a light microscope (Zeiss). Megakaryocyte spreading In vitro cultivated BM MKs of male mice were allowed to adhere and spread at 37 °C and 5% CO 2 on coverslips coated with fibrillar collagen type I (50 μg ml −1 ; Nycomed), fibrinogen (100 μg ml −1 ; F4883,Sigma-Aldrich) or CRP (6 μg ml −1 ) for the indicated time points. MK spreading was stopped by fixation and permeablization of the cells using PHEM buffer supplemented with 4% PFA and 1% IGEPAL CA-630. Immunofluorescence staining of cultured or spread MKs To visualize the cytoskeleton, the cultured MKs were spun onto glass slides (Shandon Cytospin 4, Thermo Scientific), fixed and permeabilized in PHEM buffer supplemented with 4% PFA and 1% IGEPAL CA-630, and blocked with 1% BSA in PBS. F-actin was stained using phalloidin-Atto647N (170 nM, 65,906, Fluka) and tubulin was either stained with anti-α-tubulin–Alexa F488 (3.33 μg ml −1 , 322588 (B-5-1-2), Invitrogen) or anti-acetyl–tubulin (2 μg ml −1 , sc-23950 (6-11B-1), Santa Cruz Biotechnology Inc.) antibody. Phospho-ASAP (10 μg μl −1 , 600-401-910; Rockland Inc.), WASp (10 μg μl −1 , #4860, Cell Signaling) or vinculin (4 μg μl −1 , sc-5573, Santa Cruz Biotechnology Inc.) staining served as podosome marker. Nuclei were stained using DAPI (1 μg μl −1 , D1306, Invitrogen) before mounting of samples with Fluoroshield (F6182, Sigma-Aldrich). Visualization was performed with a Leica TCS SP5 confocal microscope (Leica Microsystems). Determination of MK ploidy To determine BM MK ploidy, both femora of male mice were isolated, and the BM was flushed and homogenized. Unspecific binding sites of the 5D7 antibody were blocked by incubation of the cell suspension with 0.02 μg μl −1 anti-FcγR antibody (553,142 (2.4G2), BD Pharmingen). Afterwards, MKs were stained using a fluorescein isothiocyanate-conjugated anti-GPIIb antibody (10 μg ml −1 , 5D7). Finally, the cells were fixed, permeabilized and the DNA was stained using 50 μg ml −1 propidium iodide (P3561, Invitrogen) staining solution with 100 μg ml −1 RNaseA (EN0202, Fermentas) in PBS. Analysis was performed by flow cytometry and FlowJo software (Tree Star Inc., Ashland, USA). Data analysis The presented results are mean±s.d. from at least three independent experiments per group, if not otherwise stated. Differences between control and knockout mice were statistically analysed using the Student’s t -test. P- values<0.05 were considered as statistically significant: * P <0.05; ** P <0.01; *** P <0.001. Results with a P -value>0.05 were considered as not significant. How to cite this article: Bender, M. et al. Megakaryocyte-specific Profilin1-deficiency alters microtubule stability and causes a Wiskott–Aldrich syndrome-like platelet defect. Nat. Commun. 5:4746 doi: 10.1038/ncomms5746 (2014).